Chemical control of electrical contact tosp2carbon atoms Carbon-based nanostructures are attracting tremendous interest as components in ultrafast electronics and optoelectronics. The electrical interfaces to these structures play a crucial role for the electron transport, but the lack of control at the atomic scale can hamper device functionality and integration into operating circuitry. Here we study a prototype carbon-based molecular junction consisting of a single C 60 molecule and probe how the electric current through the junction depends on the chemical nature of the foremost electrode atom in contact with the molecule. We find that the efficiency of charge injection to a C 60 molecule varies substantially for the considered metallic species, and demonstrate that the relative strength of the metal-C bond can be extracted from our transport measurements. Our study further suggests that a single-C 60 junction is a basic model to explore the properties of electrical contacts to meso- and macroscopic sp 2 carbon structures. Thanks to their unique transport properties, carbon nanotubes (CNT), graphene sheets and nanoribbons are promising components for future nanoelectronics [1] . A close attention is paid to the connections of these graphitic structures to external metallic leads where the injection and the collection of charges are controlled [2] , [3] , [4] . Indeed, bad interfaces might ruin the transport properties of such carbon-based devices. To this respect, the chemical nature of the contacting leads is of major importance; it affects the electronic properties [5] and, depending on the reactivity, the geometry of the contact [6] . The impact of these two aspects on the transport properties is entangled and, for mesoscopic structures, it is challenging to address them separately. Exploring the evolution of these parameters for contacts shrunk to the limit of individual atoms might solve this issue. Scanning tunnelling microscopy (STM) contact experiments with fullerene molecules have revealed the decisive impact of atomic-scale modifications on transport properties [7] , [8] , [9] , [10] . Recently, some of us demonstrated that the conductance of a Cu–C 60 –Cu junction varies by more than an order of magnitude as a function of the number of Cu atoms in direct contact with the C 60 molecule [11] . For small contact sections (that is, a single-atom contact) the conductance is limited by charge injection to the molecule, and depends essentially on the electronic and geometrical properties of the metal-C atomic contact, which acts as a conductance ‘bottleneck’. Here we probe the charge injection efficiency at the interface between a C 60 molecule and single metallic atoms of different chemical nature. We demonstrate that information on the reactivity between the fullerene and each specific atom can be extracted from our experiments, which match the properties observed at the mesoscopic scale. First-principles transport simulations with a novel scheme to describe the single-C 60 junction reproduce the experimental findings and reveal how the chemical valence of the contacting atom determines the conductance of the junction [12] , [13] , [14] . Our study further demonstrates that atomic-scale junctions may be used to explore the properties of mesoscale graphitic contacts. Metal adatoms as chemically controlled electrodes To use different metal adatoms (M 1 =Cu 1 , Au 1 , Pd 1 , Fe 1 , Ti 1 , Al 1 ) deposited on a Cu(111) surface as chemically controlled electrodes for molecular contacts, the apex of our STM tip was functionalized with a C 60 molecule previously evaporated on the surface [15] . 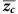Table 1 Absolute experimental contact distancesand contact conductances. No description available Figure 1a shows metallic adatoms imaged with a C 60 tip at a sample voltage corresponding to the second lowest unoccupied molecular orbital (LUMO+1) of the molecular tip. The image reveals that this particular C 60 -functionalized tip is oriented with a bond between a pentagon and a hexagon (5:6 bond) towards the substrate [16] . Depending on the chemical nature of the adatom, a varying ‘apparent height’ is exhibited in the STM images as highlighted in the close-up views in Fig. 1b–d . Figure 1: Individual metal adatoms contacted with a C 60 -functionalized STM tip. ( a ) STM image (7.0 × 6.2 nm 2 ) of different metal adatoms on Cu(111) acquired with a C 60 tip at a sample voltage V =1.7 V. ( b – d ) Close-up views (1.4 × 1.4 nm 2 ) of Cu 1 , Au 1 and Fe 1 images with a C 60 tip for tunnelling conditions corresponding to the initial parameter of the traces in f . ( e ) Sketch of the C 60 tip where z =0 corresponds to contact with the flat surface. ( f ) Experimental conductance traces G ( z ) in units of the conductance quantum G 0 =2 e 2 / h . Black crosses mark the contact points defined as the intersection of the contact and transition regimes such as indicated by the dashed grey lines in panel f for the bare surface data. Full size image Figure 1e–f show contact experiments obtained with a C 60 -terminated STM tip and the different adatoms. As expected, the conductances vary exponentially with the tip approach in the tunnelling regime (large z ). At shorter distances, a change in the slopes is observed, which marks a transition towards a contact regime. A contact distance z c and a contact conductance G c (black crosses in Fig. 1f ) are determined for each conductance trace following the method detailed in ref. 11. We emphasize that the contact measurements performed on Au 1 , Cu 1 and Fe 1 were acquired with the same C 60 tip and can be directly compared. The traces obtained on Pd 1 , Ti 1 and Al 1 pertain to other sets of measurements where they were compared with Cu 1 . Taking Cu 1 as a reference, it is therefore possible to compare data from different experiments with different adatom species. Using this method, the impact of different molecular orientations and of different tip-side interfaces between C 60 and metal on the experimental data is strongly reduced. 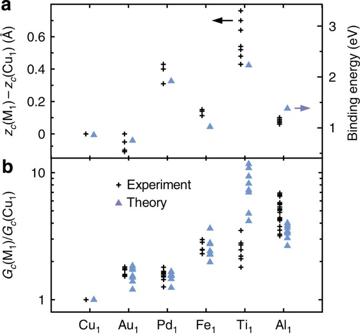Figure 2: Mechanical and conductive trends with different adatom electrodes. (a) Experimental (black crosses) contact distanceszcand (b) contact conductancesGcfor each of the considered metallic adatoms M1, obtained with different C60tips. As a common reference, the data are (a) compared with or (b) normalized by the value obtained on Cu1. In panela, the experimental contact distances are compared with calculated binding energies between an atom M1and a single C60molecule. In panelb, the experimental data are compared with calculated conductances (normalized by Cu1) for different electrode separations and binding sites (see text). The scattering in the theoretical data (blue triangles) corresponds to calculations for different lateral adatom positions and distances with respect to the C60tip. Figure 2 and Table 1 summarizes the relative distances and conductances at contact. Figure 2: Mechanical and conductive trends with different adatom electrodes. ( a ) Experimental (black crosses) contact distances z c and ( b ) contact conductances G c for each of the considered metallic adatoms M 1 , obtained with different C 60 tips. As a common reference, the data are ( a ) compared with or ( b ) normalized by the value obtained on Cu 1 . In panel a , the experimental contact distances are compared with calculated binding energies between an atom M 1 and a single C 60 molecule. In panel b , the experimental data are compared with calculated conductances (normalized by Cu 1 ) for different electrode separations and binding sites (see text). The scattering in the theoretical data (blue triangles) corresponds to calculations for different lateral adatom positions and distances with respect to the C 60 tip. Full size image Table 1 Absolute experimental contact distances and contact conductances . Full size table Mechanical aspects of contact formation First we focus on the mechanical aspects of the different junctions. Figure 2a shows that the contact takes place at different tip-sample distances z c depending on the chemical nature of the metallic adatom. For instance, the contact point occurs systematically at larger z c values with Ti 1 than with any of the other species. We find that the experimental variation in z c correlates very well with binding energies E b (blue triangles) between an atom M 1 and a single C 60 molecule calculated using density functional theory (DFT), see Methods section. The substrate has little impact on these binding energy trends, as discussed in Supplementary Fig. 1 . This suggests that the shape of the conductance trace around the point of contact is a measure of the attractive chemical forces between the adatom and the C 60 tip. Indeed, when the C 60 tip approaches the adatom, the attractive force between them increases giving rise to an elastic response [17] . The larger the attractive force between the molecule and the adatom, the ‘sooner’ a contact is established (that is, larger z c ). Our DFT-generalized gradient approximation (GGA) calculations [18] , [19] for the various junctions ( Fig. 3a ) also support that the variation observed in Fig. 2a is not due to the natural height variations of the different adatoms on Cu(111) ( Supplementary Fig. 2 ). These findings also agree with measurements of the sticking behaviour of mesoscopic metallic electrodes on single-wall CNT [6] , supporting a hierarchy E b (Pd)> E b (Fe)> E b (Al)> E b (Au) for the binding energy. Theoretical works have revealed similar hierarchies for metallic adatoms [20] , clusters of metallic atoms [5] , and metal surfaces [21] interacting with graphene sheets. While the reactivity between sp 2 carbon atoms and metallic electrodes varies with the dimensionality (0D, 1D or 2D) and the curvature of the graphitic structure, it is noticeable that our atomic-scale experiment reproduces accurately all these trends. 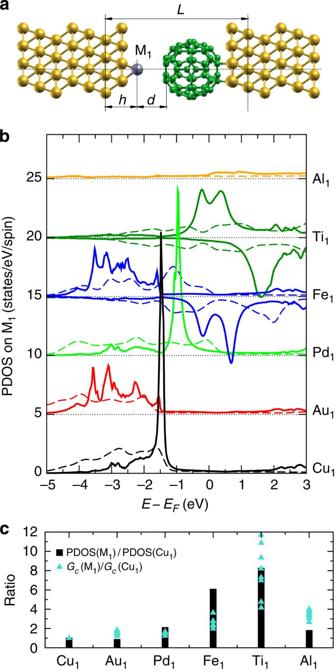Figure 3: Analysis of calculated junction properties. (a) Model of the C60–M1junctions considered in the calculations. (b) PDOS onto adatom basis (full lines: adatoms positioned in hollow sites on the molecular symmetry axis,L=18.5 Å) compared with the density of states for the same species in its bulk environment (dashed lines,Supplementary Fig. 5). For Fe and Ti, the two spin components are shown with opposite sign. The datasets are offset for clarity. (c) Comparison of adatom PDOS at the Fermi level (L=18.5 Å) with the calculated junction conductanceGc(M1) at different electrode separations, normalized with respect to Cu1. Figure 3: Analysis of calculated junction properties. ( a ) Model of the C 60 –M 1 junctions considered in the calculations. ( b ) PDOS onto adatom basis (full lines: adatoms positioned in hollow sites on the molecular symmetry axis, L =18.5 Å) compared with the density of states for the same species in its bulk environment (dashed lines, Supplementary Fig. 5 ). For Fe and Ti, the two spin components are shown with opposite sign. The datasets are offset for clarity. ( c ) Comparison of adatom PDOS at the Fermi level ( L =18.5 Å) with the calculated junction conductance G c (M 1 ) at different electrode separations, normalized with respect to Cu 1 . Full size image Chemical trends of the adatom on contact conductance We next turn to the discussion of the contact conductance values. The experimental data in Fig. 2b (black crosses) reveal that G c is on average about 1.6 times higher for Au 1 and Pd 1 than for Cu 1 contacts. The largest average ratio was observed for Al 1 . Although we took the greatest care to locate the molecular tip over each adatom with the same relative position before the tip approach, sub-angström variations of this parameter are unavoidable. Such small variations can lead to different contact geometries and, consequently, to different contact conductances [9] . This explains the scattering in the experimental data in Fig. 2b . In our simulations we account for this aspect by considering different lateral positions of the adatoms with respect to the C 60 tip [11] . We also consider different C 60 -adatom distances around the point of contact ( Fig. 3a ). The result of these simulations is displayed as blue triangles in Fig. 2b . An overall good agreement is obtained between experiment and theory. The conductance ratios are quantitatively reproduced for the Au 1 , Fe 1 and Pd 1 species. Ti 1 and Al 1 are also found to be the most conductive species, but contrary to the experiment theory assigns a larger conductance to Ti 1 than to Al 1 . Our conductance ratios also agree with simulations for metal-graphene and metal-CNT interfaces [5] , [22] . Importantly, these results confirm that the efficiency of charge injection to a C 60 molecule can vary substantially for different metal adatoms, independently of any geometrical considerations. To rationalize the observed hierarchy, it is useful to consider the projected density of states (PDOS) on the different metallic adatoms as shown in Fig. 3b and Supplementary Fig. 3 . For Cu 1 , Au 1 and Pd 1 a d -orbital adatom resonance is present significantly below the Fermi level E F . Around E F , these three species as well as Al 1 exhibit no particular spectral features corroborating that their sp electronic states of the free atoms hybridize strongly with Cu(111). The situation is very different for Fe 1 and Ti 1 which both exhibit a spin-polarized electronic structure with d -orbital resonances located around E F . For Fe 1 (Ti 1 ), the PDOS at E F is dominated by the minority (majority) spin channel, rather analogous to the case of these metals adsorbed on graphene [20] . The transmission spin polarization [23] is predicted to be as high as 88% in the case of Ti ( Supplementary Fig. 4 ). Figure 3c compares the calculated junction conductances with the PDOS( E F ) of the adatom at relatively large electrode separation ( L =18.5 Å, Fig. 3a ). To a first approximation, it is observed that the conductance is related to the PDOS. This interpretation in terms of PDOS on the adatoms also offers an explanation for the overestimated conductance of Ti 1 in the simulations. Close to resonant transport conditions—that is, when the adatom d -orbitals are nearly aligned with E F —the conductance depends sensitively on the resonance position and width. An inadequate description of the strong Coulomb repulsion between the 3 d electrons localized on the adatom with standard DFT methods (and consequently their hybridization with the substrate) can therefore have a large impact on the calculated conductance. Although theory still provides a qualitative agreement with experiment in these cases (Fe 1 and Ti 1 ), a quantitative comparison needs to be taken with caution. Figure 3b also compares PDOS of the various metal adatoms with the corresponding density of states in the bulk ( Supplementary Fig. 5 ). Interestingly, despite of very different environments, their spectral features are rather similar. The main difference is obtained for Pd, where the d -band in bulk reaches E F while it is located well below for Pd 1 on Cu(111). This general correspondence supports the notion that our single adatoms can be considered representative for meso- and macroscopic electrodes. Therefore noble metals Cu 1 and Au 1 as well as Pd 1 (closed d -shell elements) are generally less favourable for charge injection to C 60 than the open d -shell elements Fe 1 and Ti 1 or the open p -shell element Al 1 . These observations suggest that the ability of a given metal to inject charges to sp 2 carbon can, to some extent, be intuited from its chemical valence. Adatom influence on C 60 orbitals Finally, the electronic properties of the C 60 are affected by the hybridization with the different adatoms [11] , [24] with consequences for the junction conductance. 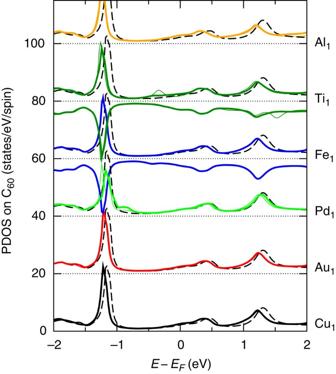Figure 4: Influence of adatoms on the C60orbitals. PDOS onto the C60basis at relatively small electrode separation (L=17.2 Å.Fig. 3a). Adatoms in hollow sites on the molecular symmetry axis (thin lines) as well as adatoms shifted one hollow site away (thick lines) are considered. For Fe and Ti, the two spin components are shown with opposite sign. The datasets are offset for clarity and compared with PDOS for the isolated C60tip (dashed black lines). Figure 4 shows the PDOS onto the C 60 basis at relatively small electrode separation ( L =17.2 Å, Fig. 3a ). It reveals the characteristic spectral features of the C 60 tip (essentially the highest occupied molecular orbital around −1.2 eV, the LUMO around 0.4 eV and the LUMO+1 around 1.2 eV), but also subtle differences depending on the adatom species. Compared with the PDOS for the isolated C 60 tip (dashed black lines), it is observed that the spectrum is only weakly perturbed by the interaction with the adatoms. For Pd 1 , Fe 1 and Ti 1, additional features appear coinciding with the d -resonances shown in Fig. 3b . The stronger impact of these adatoms on the C 60 orbitals is consistent with their significant reactivities reported in Fig. 2a . Figure 4: Influence of adatoms on the C 60 orbitals. PDOS onto the C 60 basis at relatively small electrode separation ( L =17.2 Å. Fig. 3a ). Adatoms in hollow sites on the molecular symmetry axis (thin lines) as well as adatoms shifted one hollow site away (thick lines) are considered. For Fe and Ti, the two spin components are shown with opposite sign. The datasets are offset for clarity and compared with PDOS for the isolated C 60 tip (dashed black lines). Full size image Figure 4 also reveals that the molecular resonances shift to lower energies as the contact is established, suggesting that these adatoms transfer additional electrons to C 60 (for the full evolution with electrode separation L , see Supplementary Fig. 6 ). As a consequence, the LUMO becomes more resonant with the Fermi level and conductance is enhanced. [11] These shifts are weak with Pd 1 (little charge transfer) but strong with Al 1 and Ti 1 (significant charge transfer). The differences among the adatoms may therefore affect the conductance hierarchy for larger contacts (more than one atom); for example, the conductance would be expected to increase more rapidly with the number of atoms in the cluster for Al 1 and Ti 1 than for Pd 1 . We have presented a systematic approach to probe the impact of electrode material on structure and electron transport at metal- sp 2 carbon interfaces. DFT simulations confirm our observations and rationalize the observed properties. We find that some experimental parameters (the contact distance z c ) directly reflect the strength of the metal-C bonds, but also that this strength does not necessarily reflect its conductive properties. In fact, we conclude that the ability of a metal atom to efficiently inject charges into a sp 2 carbon atom is intimately linked to its chemical valence. For transition metals, it appears that elements in the centre of the d -block present a higher ability for charge injection than atoms from the d -block extrema due to a higher density of states at the Fermi level. Charge transfer between the metal adatom and the contacted C atoms of the C 60 molecule modifies somewhat the position of the molecular resonances that also affects the conductance of the atomic-scale contact. Our single-C 60 junctions are thus good models to explore the properties of electric contacts to sp 2 carbon materials. STM setup The experiments were performed with an Omicron low-temperature STM operated at ≈4.5 K in ultrahigh vacuum (below 10 −10 mbar). Cu(111) samples and etched W tips were prepared by Ar + bombardment and annealing. W tips were indented into the sample surface to cover them with Cu. Approximately 0.2 monolayer of C 60 molecules were deposited on a sample kept at room temperature. Au, Pd, Fe, Ti or Al atoms were deposited on the C 60 -covered Cu(111) surface kept at low temperature (4.5 K). Cu atoms were deposited using the method described in ref. 25 . Identification of the different metallic species In a first step, each of the metallic species (except Cu 1 ) was evaporated individually (that is, different experimental sets) on a pristine Cu(111) sample maintained at low temperature. As referenced in the paper, Cu 1 was systematically deposited by contacting the Cu(111) surface with the STM tip. For Cu 1 , Au 1 and Fe 1 , it was possible to register constant height differential conductance (d I /d V ) spectra over a large energy range ( Fig. 5a,b ). The d I /d V spectra were acquired using lock-in detection with a modulation frequency of 740 Hz and a root-mean-square modulation amplitude of 10 mV. These data reveal resonances characteristic of the different species. The d I /d V spectra of Cu 1 /Cu(111) are even referenced in the literature [26] . Using these signatures, it was easy to discriminate these three adatoms from each other on the surface.The d I /d V spectra of Pd 1 , Ti 1 and Al 1 could not be measured because of instabilities at high voltages. This is why these elements were measured separately and were only compared with Cu 1 (which can be easily identified). It is therefore impossible to take one species for another. 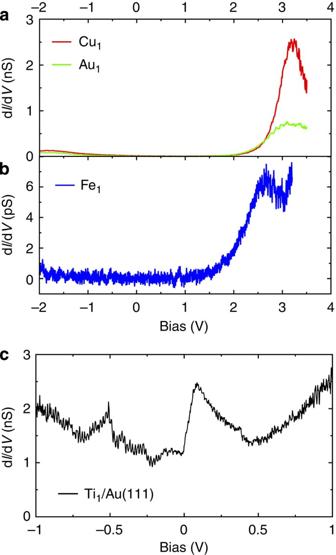Figure 5: Experimental constant-height spectra of deposited adatoms recorded with a metallic STM tip. (a) Cu1, Au1and (b) Fe1deposited on Cu(111). Note that the spectrum inbwas acquired with a lower current set point to limit instabilities at high voltages. These spectra are characteristic of the different species and are used to identify them. (c) Ti1deposited on Au(111). The same features as those reported in ref.27confirm that we evaporated Ti1. The structure around ≈−0.5 V corresponds to the localization of the Au(111) surface state at the adatom. Figure 5: Experimental constant-height spectra of deposited adatoms recorded with a metallic STM tip. ( a ) Cu 1 , Au 1 and ( b ) Fe 1 deposited on Cu(111). Note that the spectrum in b was acquired with a lower current set point to limit instabilities at high voltages. These spectra are characteristic of the different species and are used to identify them. ( c ) Ti 1 deposited on Au(111). The same features as those reported in ref. 27 confirm that we evaporated Ti 1 . The structure around ≈−0.5 V corresponds to the localization of the Au(111) surface state at the adatom. Full size image We had a particularly critical look at the Ti 1 and Al 1 cases. Although the evaporation of Cu 1 , Au 1 , Pd 1 and Fe 1 is well known and relatively easy to control, Ti 1 and Al 1 are less documented. Ti 1 was deposited by T. Jamneala et al . [27] on Au(111). In this case, d I /d V data reveal a small Kondo feature at the Fermi level as well as a characteristic feature around 150 mV (most likely a 3 d -orbital resonance). We were able to reproduce these features ( Fig. 5c ), which validates the evaporation of Ti 1 . Unfortunately, Al 1 reveals no features in d I /d V spectroscopy and this strategy can thus not be used for the identification. To investigate if the evaporated material really corresponds to individual atoms (and not clusters of atoms), we used atom manipulation techniques to form dimers Al 2 and trimers Al 3 ( Fig. 6 ). The fuzzy image in Fig. 6e is a strong indication of a dimer, similar to the Cu 2 /Cu(111) case [26] . While we cannot rule out a possible contamination of the deposited adatoms, we believe the manipulation sequence is a strong support for Al 1 . 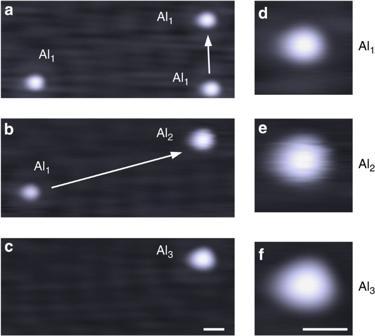Figure 6: Experimental STM images of a manipulation sequence on Cu(111). (a) Three individual Al1are arranged into (b) Al1and a dimer Al2, and finally into (c) a trimer Al3. Panels (e,f) show image close ups of the cluster to the upper right. The scale bar, 1 nm. Figure 6: Experimental STM images of a manipulation sequence on Cu(111). ( a ) Three individual Al 1 are arranged into ( b ) Al 1 and a dimer Al 2 , and finally into ( c ) a trimer Al 3 . Panels ( e , f ) show image close ups of the cluster to the upper right. The scale bar, 1 nm. Full size image C 60 –M 1 binding energy calculations The binding energy E b between a C 60 molecule and a single metallic atom M 1 is defined as E b (C 60 M 1 )= E tot (C 60 )+ E tot (M 1 )− E tot (C 60 M 1 ), where E tot ( i ) is the total energy of system i from a spin-polarized calculation. A positive binding energy thus corresponds to a stable system. DFT calculations were carried out with the Vasp code [28] using a 515-eV planewave cutoff, the generalized gradient approximation (GGA) of Perdew-Burke-Ernzerhof (PBE) for the exchange-correlation functional [29] , a tetragonal supercell of 14 × 14 × 20 Å 3 , a Gaussian smearing of 1 meV for the occupancies, and relaxations until residual forces were smaller than 0.02 eV Å −1 . Constraints were imposed to fix the metal atom to different binding sites on the C 60 cage. The results for the binding energies E b , spin magnetic moment μ and characteristic bond lengths are given in Tables 2 and 3 . These trends are mostly in agreement with those reported in ref. 23. We checked the role of applying a dipole correction for electrostatic interactions between neighbouring cells along the dimer axis, but this only affects the binding energies by a few percent for our simulation cells ( Supplementary Table 1 ). Table 2 Calculated binding energies and spin magnetic moments of C60-M 1 clusters. Full size table Table 3 Calculated bond lengths of C60-M 1 clusters. Full size table Electronic structure of model junctions The electronic structure for the various junction geometries ( Fig. 3a ) was calculated with the Siesta [18] pseudopotential DFT method with the GGA-PBE exchange-correlation functional [29] as described in refs 11 and 15 . The junctions are modelled by structures comprizing a 13-layer slab Cu(111) in a 4 × 4 representation, the adatom as well as the C 60 molecule. A standard single-zeta plus polarization basis was employed for bulk Cu (0.15-eV energy shift) and a long-ranged (0.02-eV energy shift), double-zeta plus polarization basis for C 60 and the adatoms. The pseudopotentials were constructed according to the parameters specified in Supplementary Table 2 . Real-space grid integrations were carried out using a 200 Ry energy cutoff. The 3D Brillouin zone was sampled with a 2 × 2 × 1 Monkhorst-Pack k -mesh. The lattice constant for the Cu crystal was set to 3.70 Å. As a function of varying the electrode separation L ( Fig. 3a ), the adatoms and underlying surface layer were relaxed to 0.02 eV Å −1 . The adatom heights h and radial distances r to the molecular symmetry axis are reported in Supplementary Fig. 7 . PDOS were calculated using Inelastica [30] with a 13 × 13 k || -mesh of Gauss–Kronrod points and a broadening of η =0.1 eV in the bulk part of the semi-infinite electrodes. First-principles transport simulations The electronic structure from Siesta was used to calculate the transport properties for the TranSiesta [19] setup using Inelastica [30] . The zero-bias conductance G is determined by the electron transmission function T ( E ) evaluated at the Fermi energy E F : where G 0 =2 e 2 / h is the conductance quantum. We calculate the electron transmission in two different approaches as described below. The typical approach is to calculate T ( E F ) per unit cell for a system which is periodically repeated in the plane perpendicular to the electron transport. This periodic (P) approach is consistent with the DFT treatment that relies on this periodicity. As a consequence of Bloch’s theorem, the electron transmission is averaged over k -points in the 1st Brillouin zone (with weights w k =1/ N k when using a linearly spaced mesh with N k points): Here T ( E , k ) is the electron transmission resolved in terms of electron momentum k and where the retarded Green’s function G in the device region is with S ( k ) and H ( k ) being the overlap and Hamiltonian matrices, respectively. The electrode-coupling rates are related to the self-energies via The experiment, however, concerns a single C 60 -functionalized STM tip in contact with a single adatom on Cu(111). Our alternative computational approach, more in line with this situation, corresponds to partitioning the system into periodic leads (where quantities are k -sampled) and a ‘non-periodic’ device region (which does not depend on k ). This is similar to a real-space DFT approach for STM simulations [31] , [32] and methods used for phonon transport through nanoconstrictions [33] , [34] . For our simulation cells, the natural choice is to consider the adatom and C 60 as the device, since the electronic coupling between these atoms and their periodic repetitions is significantly smaller than for the Cu atoms in the two semi-infinite electrodes. The transmission T NP ( E ) is then given by where now the device Green’s function G is thought to concern a single junction with only the self-energies being sampled over k . In practice, since the device region may not be completely decoupled from its periodic repetitions, we sample T NP ( E ) over a coarse 3 × 3- k -mesh for the device part ( H and S ) and check that there are only small variations on this mesh. 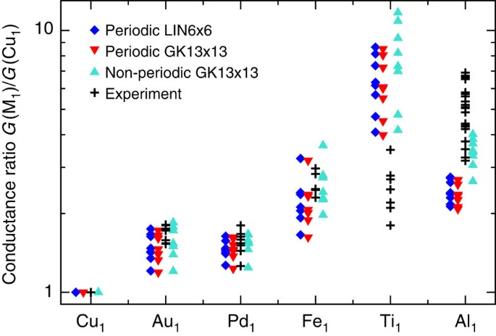Figure 7: Comparison of conductance ratios with different computational approaches. Calculations for periodic arrays of C60junctions with the transmissionT(EF) sampled on ak-mesh of 6 × 6 linearly spaced points (blue diamonds) or with 13 × 13 Gauss–Kronrod points (red triangles) in 1st Brillouin zone (1BZ). Calculations for a ‘non-periodic’ molecular junction with electrode self-energies ΣL/Rsampled on ak-mesh of 13 × 13 Gauss–Kronrod points in 1BZ (turquoise triangles). The device region consists of the adatom and C60. The experimental ratios (black crosses) are shown for comparison. Figure 7 compares the conductance ratios for the two computational schemes as well as for different sampling of k -space (6 × 6 linearly spaced points versus 13 × 13 Gauss–Kronrod points). We find that the latter ‘non-periodic’ approach, implemented on this occasion in Inelastica [30] , gives a slightly better overall agreement with the experimental conductance ratios (in particular for the Al 1 case). The figure also highlights the convergence in k -space as essentially the same conductance ratios are obtained for the two periodic sets of calculations (blue diamonds versus red triangles). In the Gauss–Kronrod scheme, a broadening of η =0.1 eV was used in the bulk electrode. Figure 7: Comparison of conductance ratios with different computational approaches. Calculations for periodic arrays of C 60 junctions with the transmission T ( E F ) sampled on a k -mesh of 6 × 6 linearly spaced points (blue diamonds) or with 13 × 13 Gauss–Kronrod points (red triangles) in 1st Brillouin zone (1BZ). Calculations for a ‘non-periodic’ molecular junction with electrode self-energies Σ L / R sampled on a k -mesh of 13 × 13 Gauss–Kronrod points in 1BZ (turquoise triangles). The device region consists of the adatom and C 60 . The experimental ratios (black crosses) are shown for comparison. Full size image The absolute conductances for both schemes are shown in Supplementary Figs 8 and 9 . Further, for the spin-polarized species (Fe and Ti) the transmission per spin channel as well as the transmission spin polarization is shown in Supplementary Fig. 4 . We also checked that the calculated conductance ratios for Al 1 shows no significant dependence on the C 60 -orientation ( Supplementary Fig. 10 ). Kondo physics We note that eventual Kondo physics [35] , [36] , beyond the DFT methods employed here, is not expected to impact our results. No Kondo resonances were experimentally resolved in d I /d V for any of the considered species on Cu(111). Therefore, even if a narrow Kondo feature would exists for species like Fe 1 and Ti 1 , it has a negligible effect on the measured conductance at V =−50 mV. How to cite this article: Frederiksen, T. et al . Chemical control of electrical contact to sp2 carbon atoms. Nat. Commun. 5:3659 doi: 10.1038/ncomms4659 (2014).